Direct observation of the spin texture in SmB6as evidence of the topological Kondo insulator Topological Kondo insulators have been proposed as a new class of topological insulators in which non-trivial surface states reside in the bulk Kondo band gap at low temperature due to strong spin–orbit coupling. In contrast to other three-dimensional topological insulators, a topological Kondo insulator is truly bulk insulating. Furthermore, strong electron correlations are present in the system, which may interact with the novel topological phase. By applying spin- and angle-resolved photoemission spectroscopy, here we show that the surface states of SmB 6 are spin polarized. The spin is locked to the crystal momentum, fulfilling time reversal and crystal symmetries. Our results provide strong evidence that SmB 6 can host topological surface states in a bulk insulating gap stemming from the Kondo effect, which can serve as an ideal platform for investigating of the interplay between novel topological quantum states with emergent effects and competing orders induced by strongly correlated electrons. Despite the great success in understanding the physical properties of topological insulators (TIs), a crucial experimental and technological problem remains unresolved—namely, most three-dimensional (3D) TI candidates are not bulk insulating [1] . The bulk conducting band, as illustrated in Fig. 1b , makes it complicated to extract the topological surface properties from transport measurements and other bulk-sensitive measurements. Furthermore, the bulk conductivity prohibits TIs from being applied as spintronic materials and from realizing exotic novel phenomena, such as Majorana fermions. Aside from this issue, at present TIs are essentially understood within non-interacting topological theory [2] , [3] ( Fig. 1b ), and thus the consequences of strong electron correlations interacting with topological phases are still unknown. 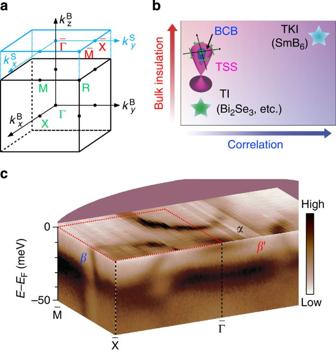Figure 1: Electronic structure of SmB6and its comparison with non-interacting TIs. (a) The first Brillouin zone of SmB6and the projection on the cleaved surface. High-symmetry points are also indicated. (b) Illustration showing the electronic correlation and bulk insulating nature of Bi2Se3and the TKI SmB6. The inset shows the electronic structure and spin texture of Bi2Se3. (c) 3D intensity plot of the photoemission data, showing the FS and electronic structure of SmB6measured with a photon energy of 26 eV and energy resolution <5 meV atT=1 K. We define the surface bands at theandpoints asαandβ, and the bulk valenced-band asγ, which are consistent with a previous study7. Figure 1: Electronic structure of SmB 6 and its comparison with non-interacting TIs. ( a ) The first Brillouin zone of SmB 6 and the projection on the cleaved surface. High-symmetry points are also indicated. ( b ) Illustration showing the electronic correlation and bulk insulating nature of Bi 2 Se 3 and the TKI SmB 6 . The inset shows the electronic structure and spin texture of Bi 2 Se 3 . ( c ) 3D intensity plot of the photoemission data, showing the FS and electronic structure of SmB 6 measured with a photon energy of 26 eV and energy resolution <5 meV at T =1 K. We define the surface bands at the and points as α and β , and the bulk valence d -band as γ , which are consistent with a previous study [7] . Full size image Recent theoretical investigations [4] , [5] , [6] have suggested that some Kondo insulators such as SmB 6 , in which electrons are strongly correlated, can possibly host non-trivial topological surface states (TSS) atop truly insulating bulk crystals, forming a special group of TIs known as topological Kondo insulators (TKIs). Our previous high-resolution angle-resolved photoemission spectroscopy (ARPES) study [7] has revealed that two-dimensional surface states reside within the Kondo band gap (Δ~20 meV relative to chemical potential) and form three Fermi surfaces (FSs) in the first surface Brillouin zone (SBZ): one is centred at the SBZ ( point in Fig. 1a ) and two (viewed as four half-FSs) encircle the midpoints of the SBZ boundaries ( points) ( Fig. 1c ). The odd number of surface bands crossing the Fermi level ( E F ) fulfills a necessary condition of TSS, and the observed surface state dispersions are in good agreement with theoretical calculations indicating that SmB 6 could be a TKI. Our observations are also consistent with transport results [8] , [9] , [10] , [11] , [12] , [13] , [14] , [15] and supported by other ARPES [16] , [17] , [18] studies, as well as scanning tunnelling microscopy measurements [19] . On the other hand, the in-gap states have also been discussed as topologically trivial polar surface states [20] , and even as bulk states [21] . Until now, there has been no conclusive evidence indicating that SmB 6 is a TKI. Therefore, identifying the topologically non-trivial nature of the in-gap states of SmB 6 is crucial for distinguishing these different explanations and verifying whether SmB 6 is indeed the first realization of a TKI. Using spin-resolved ARPES (SARPES), here we investigate the spin texture of the surface states around the points in the SBZ of SmB 6 . We show that the surface states are spin polarized with strong k || dependence. The spin-helical structure fulfills the requirement of time-reversal symmetry (TRS). Our results give direct evidence that SmB 6 is the first realization of a strongly correlated TKI. Spin polarization of the TSS along the direction In Fig. 2b , we plot the near- E F spin-integrated ARPES intensity and a momentum distribution curve (MDC) at E SR (10 meV above E F ) along the direction. The momentum cut in the SBZ is indicated by the red line (C1) in the FS mapping ( Fig. 2a ). The spin-integrated ARPES data shown in Fig. 2a,b are taken with hν =26 eV ( k z =4 π for the bulk states) at the same experimental station as the SARPES data discussed in the following. The sample temperature for the spin-integrated and SARPES measurements is 20 K, at which the Kondo gap is fully opened and the surface states dominate near E F [7] , [15] , [16] , [17] , [18] , [19] . Inside the Kondo band gap, the α - and β -surface state bands are visible in the intensity plot, which are also clearly seen as peaks of the MDC at E SR . Photon energy-dependent measurements have shown that these bands do not disperse in k z , the momentum along the surface normal, and thus are true surface states [7] , [16] , [17] , [18] . To determine the spin polarization of the surface bands, we performed spin-resolved MDC measurements along the cut (C1) at E SR . The purpose of choosing the MDC to lie at E SR is to minimize the contribution of the bulk f and d states located at E B ≥20 meV due to the limited energy resolution in spin-resolved mode (see Methods). At the same time, the count rate still allows us to acquire data with sufficient statistics in the SARPES measurements. 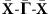Figure 2: Spin polarization of topological Dirac surface states along thedirection. (a) FS map of SmB6. (b) Low energy excitations nearEFalong the high-symmetry line. The location in thekx–kyplane is indicated by C1 ina. The red curve is the MDC atESR(10 meV aboveEF). (c) Measured spin-resolved intensity projected on thexdirection for the surface states atESR. The red and blue symbols are the intensity of spin-up and spin-down states, respectively. (d) Spin polarization along thexdirection for the surface states measured at theESR. The red and blue colour regions represent positive and negative spin polarizations (spin-up and spin-down), respectively. The black and orange arrows represent the spin polarization directions of theβ-andβ′-bands along thexaxis, respectively. (e,f) Same asc,dbut along theydirection. (g,h) Same asc,dbut along thez(out-of-plane) direction. All the results in Fig. 2 are measured with a photon energy of 26 eV and right-hand circular polarization (C+). Figure 2c,e,g shows the spin-resolved MDC intensity I ↑↓ x , y , z in the x , y and z directions, respectively, measured with hν =26 eV and right-hand circularly polarized light (C+). The in-plane spin polarization x and y axes are defined along each direction ( x and y as indicated in the coordinate system in Fig. 2a ), and the out-of-plane spin polarization z axis is along the sample normal k z . As shown in Fig. 2c,d , there is a clear difference in I ↑ x and I ↓ x at each of the two MDC main peaks that correspond to two branches of the β -bands, indicating that the surface state bands are spin-polarized along the x direction. We have also observed two more peaks between the main β -band peaks in the spin-polarization spectrum along the x direction ( Fig. 2d ). These are ascribed to the β ′-band ( Fig. 1c ), which results from the folding of β due to a surface reconstruction assuming a single domain [7] , [17] . We notice that the β ′-band is hardly resolved from the β -band in the spin-integrated spectra ( Fig. 2b ) due to the limited resolution. However, it can be observed clearly in the spin-resolved spectra because of the different spin polarization. Combining the SARPES data in Fig. 2 , we can summarize that near E F the β- and β ′-bands measured along C1 are both polarized in the x direction, as indicated by the coordinate system in Fig. 2a . Moreover, each of the pairs of β- and β ′-states located at k and -k have opposite spin polarizations, consistent with the behaviour of a spin-split Kramers pair, in accordance with TRS. Figure 2: Spin polarization of topological Dirac surface states along the direction. ( a ) FS map of SmB 6 . ( b ) Low energy excitations near E F along the high-symmetry line . The location in the k x – k y plane is indicated by C1 in a . The red curve is the MDC at E SR (10 meV above E F ). ( c ) Measured spin-resolved intensity projected on the x direction for the surface states at E SR . The red and blue symbols are the intensity of spin-up and spin-down states, respectively. ( d ) Spin polarization along the x direction for the surface states measured at the E SR . The red and blue colour regions represent positive and negative spin polarizations (spin-up and spin-down), respectively. The black and orange arrows represent the spin polarization directions of the β- and β ′-bands along the x axis, respectively. ( e , f ) Same as c , d but along the y direction. ( g , h ) Same as c , d but along the z (out-of-plane) direction. All the results in Fig. 2 are measured with a photon energy of 26 eV and right-hand circular polarization (C+). Full size image Spin polarization of the TSS along high symmetry lines To determine the spin texture of the FS pockets, we have carried out SARPES measurements along the cuts C1–C4, as indicated in Fig. 3a , using C+ polarized light and photon energies of hν =26 and 30 eV. For both photon energies, a consistent spin texture was obtained. As shown in Fig. 3c , the spin polarization (MDC at E SR ) measured with hν =30 eV along C1 is essentially the same as that in Fig. 2d taken with hν =26 eV. 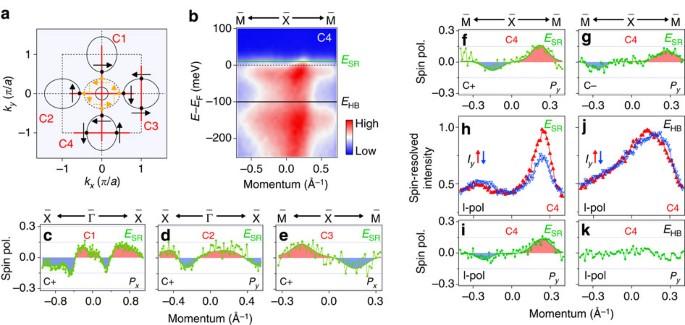Figure 3: Spin polarization of topological Dirac surface states along high-symmetry lines. (a) Schematic showing the FS of the topological surface states in SmB6, with red lines indicating the locations of spin measurements in thekx–kyplane, labelled as C1, C2, C3 and C4. The circle at the BZ centrepoint and ellipses at the middle points of BZ boundaries (points) indicate the FSs of theα- andβ-bands, respectively7,17. The dashed line ellipse at thepoint indicates the folded bandβ′7,17. The dots are thekFpositions of the bands and the arrows are the measured spin polarizations at the positions of the dots. The black dashed lines indicate the first SBZ. (b) Low-energy excitations nearEFalong the high symmetry line, measured with photon energyhν=30 eV and C+ polarization. The location in thekx–kyplane is indicated by C4 ina. (c) Spin polarization measured athν=30 eV along thexdirection for the surface states atESR(10 meV aboveEF). The location in thekx–kyplane is indicated by C1 ina. (d) Analogous toc, but for C2, where the spin polarization direction is alongy. (e) Analogous toc, but measured athν=26 eV for C3, where the spin polarization direction is alongx. (f) Analogous toc, but for C4, where the spin polarization direction is alongy. For (c–f), the photon polarization is C+. (g) Same asf, but with C– photon polarization. (h) Measured spin-resolved intensity along theydirection for the surface states atESR, measured athν=30 eV with linear light polarization. The red and blue symbols are the intensity of spin-up and spin-down states, respectively. The location in thekx–kyplane is indicated by C4 ina. (i) Spin polarization along theydirection for the surface states at theESR. (j,k) Same ash,ibut for the bulk states at higher binding energy illustrated byEHBinb. Figure 3d shows the spin polarization along C2 (perpendicular to C1). Similar to the observation along C1, the β- and β ′-bands are spin polarized, but now along the y direction. At the two k F points on cut C3 (C4), the spin polarizations of the β -band are opposite along the x ( y ) direction ( Fig. 3e,f ). The determined spin texture is summarized in Fig. 3a with spin polarizations marked by arrows. The measured spin texture, wherein the spin polarization is locked to the momentum, is fully consistent with TSS in the sense that it obeys both TRS and the crystal symmetry. This is further supported by the fact that the folded band β ′ has the same spin texture as the original band β , as expected from a simple Umklapp mechanism [22] . Figure 3: Spin polarization of topological Dirac surface states along high-symmetry lines. ( a ) Schematic showing the FS of the topological surface states in SmB 6 , with red lines indicating the locations of spin measurements in the k x –k y plane, labelled as C1, C2, C3 and C4. The circle at the BZ centre point and ellipses at the middle points of BZ boundaries ( points) indicate the FSs of the α - and β -bands, respectively [7] , [17] . The dashed line ellipse at the point indicates the folded band β ′ [7] , [17] . The dots are the k F positions of the bands and the arrows are the measured spin polarizations at the positions of the dots. The black dashed lines indicate the first SBZ. ( b ) Low-energy excitations near E F along the high symmetry line , measured with photon energy hν =30 eV and C+ polarization. The location in the k x – k y plane is indicated by C4 in a . ( c ) Spin polarization measured at hν =30 eV along the x direction for the surface states at E SR (10 meV above E F ). The location in the k x – k y plane is indicated by C1 in a . ( d ) Analogous to c , but for C2, where the spin polarization direction is along y . ( e ) Analogous to c , but measured at hν =26 eV for C3, where the spin polarization direction is along x . ( f ) Analogous to c , but for C4, where the spin polarization direction is along y . For ( c – f ), the photon polarization is C+. ( g ) Same as f , but with C– photon polarization. ( h ) Measured spin-resolved intensity along the y direction for the surface states at E SR , measured at hν =30 eV with linear light polarization. The red and blue symbols are the intensity of spin-up and spin-down states, respectively. The location in the k x – k y plane is indicated by C4 in a . ( i ) Spin polarization along the y direction for the surface states at the E SR . ( j , k ) Same as h , i but for the bulk states at higher binding energy illustrated by E HB in b . Full size image Photon polarization-dependent SARPES results It has been shown that a spin polarization signal can also appear in the photoemission process from states that possess no net spin polarization [23] . This so-called photoemission effect is discussed, for instance, for the core-level photoelectrons from non-magnetic solids [24] , the bulk valence bands of TIs [25] , as well as the bulk f states of SmB 6 (ref. 26 ). In contrast to the intrinsic spin signal from the spin-polarized initial states, the non-intrinsic spin signal caused by the photoemission effect depends on the incident photon energy and polarization. For example, the non-intrinsic spin polarization of the f states in SmB 6 caused by the photoemission effect changes direction when the photon polarization changes from C+ to left-hand circularly polarized light (C-), and vanishes with linear polarization (l-pol) [26] . The consistent momentum-locked spin texture obtained with different photon energies ( Figs 2 and 3 ) in our experiments provides evidence that the observed spin polarizations are intrinsic to the spin-polarized initial states. To rule out the possibility that the detected spin texture results from the polarization of the incident light, we conducted spin-resolved measurements using incident light with all available polarizations. Figure 3f,g,i shows the results along C4 detected by using C+, C− and linear polarizations of the incident light. The same spin polarizations from differently polarized light give further confidence that the observed spin polarizations reflect the intrinsic spin structure of the initial states. No spin polarization of the bulk states As any spin polarization of the bulk f states caused by a photoemission effect should be vanish with linearly polarized light [26] , the results obtained with the linearly polarized light ( Fig. 3h,i ) further indicate that the spin polarization originates from the surface β -band, and not from contamination of the bulk f states due to the limited energy resolution used in SAPRES measurements. To further exclude contamination from the bulk d states as an origin of the observed spin polarizations of the MDCs studied at E SR , we performed measurements at a higher binding energy ( E HB as illustrated in Fig. 3b ), where the bulk d states dominate the photoemission intensity. Figure 3j,k shows the spin-resolved MDC intensity I ↑↓ and the spin polarization spectra along the y direction, taken with linearly polarized light (l-pol). In contrast to the spectra at E SR ( Fig. 3h,i ), the spin-resolved MDCs at E HB show negligible difference, indicating that the photoelectrons from the spin-degenerate bulk d -states are not spin polarized. Therefore, we conclude that the spin signal at E SR is dominated by the surface states, which provides compelling evidence that SmB 6 is the first realization of a TKI. 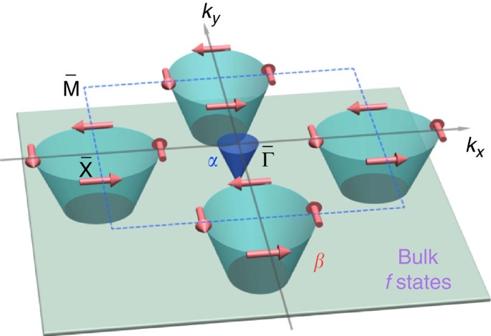Figure 4: Schematic of the spin-polarized surface state dispersion in the TKI SmB6. The blue and green curved surfaces centred at theandpoints represent theα- andβ-bands, respectively. The plane sitting below represents the bulkfstates. The spin polarizations of theβ-band are indicated with red arrows. The shape and size of theα-band are from refs7,17. The blue dashed lines indicate the first SBZ. Figure 4 schematically summarizes our main experimental finding of the spin structure of the surface bands of SmB 6 . For simplicity, we consider the situation without folding bands. The spin orientations of the electrons in the in-gap surface β- band, which is located between the strongly localized bulk f states and the chemical potential, are locked to their momenta; namely, at opposite momenta ( k and -k ), the surface states have opposite spins. This anti-clockwise spin texture for the surface band in SmB 6 shows a great similarity to other 3D TIs (Bi 2 Se 3 , Bi 2 Te 3 , etc. ), which each has a FS from a single pocket centred at the point in the SBZ [27] , [28] . Extensive ARPES studies have shown that SmB 6 has a surface FS formed by three electron pockets with Kramers points located around the SBZ centre and boundary [7] , [16] , [17] . The revealed spin texture, together with the odd number of pockets, is consistent with the metallic states at the surface of SmB 6 being non-trivial topological surface states, and the findings here strongly support recent theoretical predictions that SmB 6 is a TKI [5] , [5] , [6] . A crucial and so far unresolved problem for the real-world implementation of TIs is that most 3D TI candidates are not bulk-insulating [4] , [29] . On the other hand, SmB 6 is a mixed valence Kondo insulator. Owing to the hybridization of the nearly localized 4 f bands with the dispersive conduction band, a band gap opens near the chemical potential at low temperature, leading the system in to a good bulk insulator [4] , [30] , [31] , [32] . Thus, the direct identification of SmB 6 as a TKI is a significant advance in realizing a topological quantum state of matter in which the metallic edge states, protected by TRS, are located on a true bulk insulator. It is also worthwhile to mention that the metallic TSS formed by the electron pockets at low temperatures can provide a natural explanation for the longstanding puzzle that the resistivity in SmB 6 saturates to a finite value instead of being divergent [30] , [31] , [32] . Meanwhile, the coexistence of the topological surface states and the strongly correlated bulk states offers new opportunities for understanding TIs beyond the non-interacting topological theory. Figure 4: Schematic of the spin-polarized surface state dispersion in the TKI SmB 6 . The blue and green curved surfaces centred at the and points represent the α - and β -bands, respectively. The plane sitting below represents the bulk f states. The spin polarizations of the β -band are indicated with red arrows. The shape and size of the α -band are from refs 7 , 17 . The blue dashed lines indicate the first SBZ. Full size image (S)ARPES measurements SARPES and ARPES measurements were performed at the Surface/Interface Spectroscopy beamline at the Swiss Light Source with the COPHEE station. The two orthogonally mounted 40 kV classical Mott detectors allow for the determination of all three components of the spin of the electron ( P x , P y and P z ) as a function of its energy and momentum [33] , [34] . To achieve this, the spin polarization curves obtained for the three spatial directions are fitted simultaneously with the sum of all the Mott channels, that is, the spin integrated signal. Further technical details of the data acquisition and analysis can be found in ref. 35 . The SARPES measurements were repeated for several samples with photon energies ranging from 26 to 30 eV and with circular and linear light polarizations. Results with different photon energies and light polarizations are consistent. All the spin-integrated and spin-resolved data shown in Figs 2 and 3 are taken at T =20 K, where the Kondo gap is fully open [7] , [15] , [16] , [17] , [18] . The energy and angle resolutions were 60 meV (full width at half maximum) and 3% of the SBZ, respectively, to allow for acceptable statistics. Because of the low photoemission signal, the typical duration of a spin-resolved MDC was about 6 h. After this period, the sample quality was confirmed again by spin-integrated measurements. Clean surfaces for the (S)ARPES measurements were obtained by cleaving the crystals in situ at low temperature (20 K) in a working vacuum better than 2 × 10 −10 mbar. Shiny mirror-like surfaces were obtained after cleaving the samples, confirming their high quality. Sample fabrication High-quality single crystals of SmB 6 were obtained by growth from Al-flux using samarium pieces (99.9%), boron powder (99.99%) and aluminum pieces in a ratio of 0.5 g of Sm:B (1:6) and 50 g of Al (99.99%). The growth was done in a vertical gradient furnace under continues argon flow at a temperature up to 1,500 °C with a cooling rate of 5 K h −1 . The aluminum flux was removed by potassium hydroxide solution. The crystals, which are millimetre sized, have a bar shape, black colour and flat, mirror-like surfaces. How to cite this article: Xu, N. et al. Direct observation of the spin texture in SmB 6 as evidence of the topological Kondo insulator. Nat. Commun. 5:4566 doi: 10.1038/ncomms5566 (2014).